Arabidopsis NIN-like transcription factors have a central role in nitrate signalling In plants, nitrate is not only a major nitrogen source but also a signalling molecule that modulates the expression of a wide range of genes and that regulates growth and development. The critical role of nitrate as a signalling molecule has been established for several decades. However, the molecular mechanisms underlying the nitrate response have remained elusive, as the transcription factor that primarily responds to nitrate signals has not yet been identified. Here we show that Arabidopsis NIN-LIKE PROTEIN (NLP) family proteins bind the nitrate-responsive cis -element and activate nitrate-responsive cis -element-dependent and nitrate-responsive transcription. Our results also suggest that the activity of NLPs is post-translationally modulated by nitrate signalling. Furthermore, the suppression of NLP function impairs the nitrate-inducible expression of a number of genes and causes severe growth inhibition. These results indicate that NLPs are the transcription factors mediating the nitrate signal and thereby function as master regulators of the nitrate response. Nitrogen is a primary macronutrient that is required in abundance in plants. As most land soils globally are nitrogen-deficient, and nitrate, which is a major nitrogen source for land plants readily flows into aquatic ecosystems, land plants need to adapt their growth and metabolism in response to fluctuations in nitrogen availability [1] , [2] , [3] , [4] , [5] , [6] , [7] , [8] . Nitrate is a key signalling molecule that regulates this adaptation process. Nitrate modulates the expression of a wide spectrum of genes, including not only nitrate assimilation-associated genes such as nitrate reductase ( NR ) genes and nitrite reductase ( NIR ) genes, but also genes involved in other metabolic pathways and some developmental processes [9] , [10] , [11] , [12] . As the nitrate-inducible modulation of these genes occurs even in mutants lacking NR activity, nitrate itself is believed to be a signalling molecule [1] , [13] . Furthermore, because primary nitrate-induced gene expression does not require de novo protein synthesis [11] , [14] , [15] , nitrate likely activates a pre-existing but as yet unidentified transcription factor post-translationally, and then actuates nitrate response mechanisms. In several past studies, regulatory genes involved in nitrate signalling and response pathways have been characterized. For instance, an Arabidopsis MADS-box gene, ANR1 , has been shown to promote the lateral root growth on nitrate-rich patches [2] , [16] , [17] . Another Arabidopsis gene for NSR1, which is structurally close to the PHR1 transcription factor that functions in phosphorus starvation responses, has been identified as a nitrogen starvation-inducible gene [18] . Furthermore, phenotypic analysis of Arabidopsis mutants has revealed that the disruption of one of the NIN-LIKE PROTEIN genes ( NLP7 ) produced features of nitrogen-starved plants, accompanied by impaired expression of genes for nitrate transporter and NR [19] . As NIN, which is necessary for symbiosis between legumes and nitrogen fixing bacteria, had been proposed as a putative transcription factor [20] , NLP7 is also speculated to be a regulatory protein associated with nitrogen assimilation. The LBD genes are also proposed to encode transcription factors associated with nitrate-responsive gene expression, because overexpression of LBD37, LBD38 or LBD39 represses the expressions of nitrate transporter and NR genes in Arabidopsis [21] . Another Arabidopsis gene, GNC , has also been identified as a nitrate-inducible gene encoding a putative transcription factor of the GATA family [22] . In addition to these putative transcription factors, two Arabidopsis proteins, NRT1.1 dual-affinity nitrate transporter and CIPK8 protein kinase, have also been suggested to have roles in nitrate response as a nitrate sensor [23] and a regulator in the presence of high concentrations of nitrate [24] , respectively. Although an increasing number of factors involved in nitrate signalling and response has been identified, the key factor in the mechanism for nitrate response, namely the transcription factor that primarily responds to nitrate signalling, has not yet been identified. Nitrate-responsive transcription factors have been identified in bacteria, fungi and algae [25] , [26] , [27] . However, no protein in higher plants is similar to the nitrate-responsive transcription factors in these organisms, suggesting that different factors might mediate nitrate signalling in higher plants. In our present study, to identify transcription factors responsible for the primary nitrate induction of gene expression in plants, we performed yeast one-hybrid (Y1H) screening using a 43-bp sequence, which was previously identified as an authentic nitrate-responsive cis -element (NRE) conserved in NIR gene promoters from various higher plants [28] , [29] . The results of our analyses indicate that NLPs are NRE-binding proteins with transcriptional activator roles that convert nitrate signals to transcriptional regulation events, and that function in the nitrate-regulated expression of many genes in Arabidopsis. Identification of NLPs as NRE-binding proteins To identify transcription factors that interact with NREs, we performed Y1H screening using a HIS3 reporter gene under the control of four copies of NRE (4 × NRE) and Arabidopsis complementary DNA (cDNA) libraries ( Fig. 1a ). We thereby identified 13-positive cDNA clones, all of which encompassed DNA sequences for the RWP-RK domain of NLPs ( Supplementary Table S1 ). 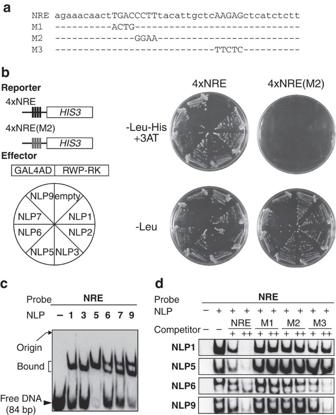Figure 1: Binding of the RWP-RK domain of NLPs to the NRE ofNIR1. (a) Sequences of the wild-type and mutated NREs used in the Y1H (b) and EMSA (c,d) experiments. (b) Y1H assay. Yeast harbouring the4 × NRE-HIS3or4 × NRE(M2)-HIS3reporter gene were transformed with expression vectors for the GAL4 activation domain fused to the RWP-RK domain of the indicated NLPs, and grown on control (-Leu) and selection medium (-Leu-His+15 mM 3-aminotriazole). (c) EMSA analysis using the wild-type NRE as a probe and recombinant RWP-RK domains of the indicated NLPs. (d) EMSA analysis in which non-labelled wild-type and mutated NREs were used as competitor DNA at an excess molar ratio (+, 1:5; ++, 1:25). Figure 1: Binding of the RWP-RK domain of NLPs to the NRE of NIR1 . ( a ) Sequences of the wild-type and mutated NREs used in the Y1H ( b ) and EMSA ( c , d ) experiments. ( b ) Y1H assay. Yeast harbouring the 4 × NRE-HIS3 or 4 × NRE(M2)-HIS3 reporter gene were transformed with expression vectors for the GAL4 activation domain fused to the RWP-RK domain of the indicated NLPs, and grown on control (-Leu) and selection medium (-Leu-His+15 mM 3-aminotriazole). ( c ) EMSA analysis using the wild-type NRE as a probe and recombinant RWP-RK domains of the indicated NLPs. ( d ) EMSA analysis in which non-labelled wild-type and mutated NREs were used as competitor DNA at an excess molar ratio (+, 1:5; ++, 1:25). Full size image RWP-RK is a putative DNA-binding domain, which was previously proposed in the primary structure of NIN [20] and the name of which originates from the RWP × RK motif conserved in NIN, algal minus dominance proteins [30] and five Arabidopsis proteins [20] . However, there is no experimental evidence for the binding of the RWP-RK domain to DNA. We, therefore, further characterized DNA-binding of NLPs in our present experiments. Phylogenic analysis has indicated previously that the nine Arabidopsis NLPs can be classified into three groups (NLP1 to NLP5; NLP6 and NLP7; NLP8 and NLP9), although all NLPs are highly homologous to each another and possess both the RWP-RK domain and additionally conserved amino-acid motifs [31] . Although NLP8 and NLP9 cDNAs were not isolated in our screening ( Supplementary Table S1 ), we also examined the binding of the RWK-RK domain of NLP9, and of the other NLPs, to the NRE using Y1H assays ( Fig. 1b ). The results indicate that all RWK-RK domains analysed bind to the NRE in yeast, suggesting that all NLPs may bind to this element. The NRE is a pseudopalindromic sequence comprising two half-sites separated by a 10-bp spacer sequence ( Fig. 1a ). Both sites are necessary for full nitrate induction of the expression of Arabidopsis NIR gene ( NIR1 ) in planta , although the distal half site has the dominant role [28] . We, therefore, investigated the binding specificity of NLPs using a panel of NREs with mutations within either the distal (M1 and M2) or proximal (M3) half-site ( Fig. 1a ) using electrophoretic mobility shift assays (EMSA). Consistent with the results of our Y1H assays, the RWK-RK domain of all NLPs analysed bound to the wild-type NRE in the EMSA experiments ( Fig. 1c ). However, none of the NLPs tested bound to the M2 NRE in yeast ( Fig. 1b ). Consistently, unlike the wild-type NRE, the M1 and M2 NREs did not compete with a labelled NRE probe during complex formation with any NLP. On the other hand, the M3 NRE hampered the complex formation of NLP6 and NLP9 but not that of NLP1 and NLP5 ( Fig. 1d ). Hence, all NLPs are likely to bind the NRE in a sequence-specific manner but display different requirements for the half-sites within this motif. We previously showed that a 3.7-kb sequence in the 3′-flanking region of an Arabidopsis NR gene, NIA1 , is responsible for the nitrate induction of NIA1 expression [32] . We, therefore, also tested the binding of NLP6 to several DNA fragments from the 3.7-kb region and found that NLP6 bound to two independent DNA fragments containing NRE-like sequences in vitro ( Supplementary Fig. S1a,b ). Mutational analysis indicated that at least one of these NRE-like sequences, which we designated NIA1-NRE1, functioned as an NRE ( Supplementary Fig. S1c–e ). Hence, NLPs may also regulate nitrate-inducible NIA1 expression through their interaction with NIA1-NRE1 in the 3′-flanking region of NIA1 . Taken together, our results suggest that NLPs are DNA-binding proteins that recognize NREs present in either the 5′ or 3′-flanking regions of nitrate-responsive genes [28] , [32] . NLPs are transcriptional activators NIN and NLPs had been speculated to be transcription factors due to their putative DNA-binding domains [20] . However, no evidence for this has thus far been presented. We, therefore, examined the activity of NLPs as transcription factors using an Arabidopsis protoplast transient assay system [33] , [34] . All of the tested NLPs successfully transactivated a promoter in which a 4 × NRE construct was placed upstream of the CaMV 35S minimal promoter ( Fig. 2a ). The transcriptional activation function of the NLPs was further characterized using NLP6, likely to be one of the most abundant of these proteins ( Supplementary Table S1 ). NLP6 activated the 4 × NRE promoter but not the nitrate non-inducible CaMV 35S promoter ( Fig. 2b ). NLP6 also activated the wild-type NIR1 promoter but not its M1 and M2 variants harbouring mutations within the distal half-site of the NRE. The M3 variant, in which the proximal half-site of the NRE is disrupted, was found to be marginally activated by NLP6 ( Fig. 2c ). These results indicate that NLP6, and likely also other NLPs, activate transcription via a specific interaction with the NRE. 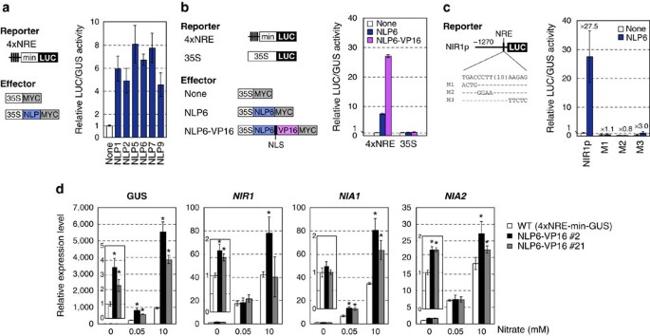Figure 2: Activation of NRE-mediated transcription by NLPs. (a) Activation of an NRE-containing promoter by NLPs in protoplast transient assays. The indicated reporter construct and effector constructs for expression of respective NLPs were co-transfected into mesophyll protoplasts that were prepared from mature leaves of Arabidopsis grown in soil for 3 weeks. (b) Stronger activation of the NRE-containing promoter by NLP6-VP16 protein in protoplast transient assays. The 35S promoter was used as a negative control. (c) Different activation of the wild-typeNIR1promoter (NIR1p) and its variants (M1-3 promoters) by NLP6 in protoplast transient assays. Mutations introduced into the NRE of theNIR1promoter are also shown. In all transient assays, an internal control plasmid (UBQ10-GUS) was co-transfected into Arabidopsis protoplasts to normalize the LUC reporter activity levels. Relative LUC activity is shown ina–c, and activation folds are also indicated inc. 4 × NRE, four copies of NRE; min, the 35S minimal promoter; 35S, the full-length 35S promoter; MYC, a sequence encoding the c-Myc epitope tag; NLS, nuclear localization signal; VP16, the transcriptional activation domain of VP16. Each construct contained the NOS terminator but it is not shown. (d) Levels ofGUS,NIR1,NIA1andNIA2transcripts in two independent lines in which NLP6-VP16 was expressed under the control of the 35S promoter. Nitrogen-starved seedlings were treated with different concentrations of nitrate for 1 h. Inserts show the transcripts levels in the seedlings treated with water. As the background line was the 4 × NRE-min-GUS line, the line is indicated by ’WT‘. Values are the means±s.d. (n=3) ina–d. *P<0.05 by two-tailed Student’st-test ind. Figure 2: Activation of NRE-mediated transcription by NLPs. ( a ) Activation of an NRE-containing promoter by NLPs in protoplast transient assays. The indicated reporter construct and effector constructs for expression of respective NLPs were co-transfected into mesophyll protoplasts that were prepared from mature leaves of Arabidopsis grown in soil for 3 weeks. ( b ) Stronger activation of the NRE-containing promoter by NLP6-VP16 protein in protoplast transient assays. The 35S promoter was used as a negative control. ( c ) Different activation of the wild-type NIR1 promoter (NIR1p) and its variants (M1-3 promoters) by NLP6 in protoplast transient assays. Mutations introduced into the NRE of the NIR1 promoter are also shown. In all transient assays, an internal control plasmid (UBQ10-GUS) was co-transfected into Arabidopsis protoplasts to normalize the LUC reporter activity levels. Relative LUC activity is shown in a – c , and activation folds are also indicated in c . 4 × NRE, four copies of NRE; min, the 35S minimal promoter; 35S, the full-length 35S promoter; MYC, a sequence encoding the c-Myc epitope tag; NLS, nuclear localization signal; VP16, the transcriptional activation domain of VP16. Each construct contained the NOS terminator but it is not shown. ( d ) Levels of GUS , NIR1 , NIA1 and NIA2 transcripts in two independent lines in which NLP6-VP16 was expressed under the control of the 35S promoter. Nitrogen-starved seedlings were treated with different concentrations of nitrate for 1 h. Inserts show the transcripts levels in the seedlings treated with water. As the background line was the 4 × NRE-min-GUS line, the line is indicated by ’WT‘. Values are the means±s.d. ( n =3) in a – d . * P <0.05 by two-tailed Student’s t -test in d . Full size image Enhancement of NLP activity promotes nitrate-inducible gene expression To further assess the role of NLPs in nitrate-inducible gene expression in planta , we employed NLP6 fused to the transcriptional activation domain of VP16 (NLP6-VP16), as this protein acts as a stronger transcriptional activator during NRE-dependent transcription in protoplasts ( Fig. 2b ). By transformation of a transgenic line harbouring the GUS reporter gene under the control of the 4 × NRE promoter (4 × NRE-min-GUS line) [28] , we generated transgenic Arabidopsis lines expressing NLP6-VP16 under the control of the 35S promoter ( Fig. 2d and Supplementary Fig. S2 ). These transformed lines still retained the ability to direct nitrate-inducible GUS expression ( Fig. 2d ). However, the expression levels of GUS were elevated in these lines. Similarly, the transcript levels of the endogenous nitrate-inducible genes, NIR1 and NR genes ( NIA1 and NIA2 ), tended to be higher in these transgenic lines, indicating that NLP6-VP16 enhances nitrate-induced gene expression in planta . Although this enhancement was small, probably because of strong activity of endogenous NLPs, it was statistically confirmed. The N-terminal region of NLP6 receives nitrate signals The results of previous reports have suggested that primary nitrate induction of gene expression does not require de novo protein synthesis [11] , [14] , [15] . Consistent with this hypothesis, NRE-dependent transcriptional activation has also been suggested to be triggered through the post-translational activation of the protein interacting with NRE in planta [29] . Because no Arabidopsis NLP gene was significantly induced by nitrate treatment ( Supplementary Fig. S3 ) and the constitutive expression of NLP6-VP16 using the 35S promoter did not lead to the constitutive activation of nitrate-inducible genes ( Fig. 2d ), we speculated that the post-translational activation of NLPs by nitrate might be the primary step for nitrate-induced gene expression. We evaluated this hypothesis by identifying the nitrate-responsive region of NLP6 using recombinant transcription factors that contained the RWP-RK domain or other regions of NLP6. The expression of the RWP-RK domain alone suppressed NRE-dependent transcription in protoplasts ( Fig. 3a ), probably because it acted as a competitive inhibitor against endogenous NLPs. In contrast, the RWP-RK domain fused to two or five copies of the VP16 transcriptional activation domain (RWPRK-VP32 and RWPRK-VP80) enhanced NRE-dependent transcription ( Fig. 3a ). Hence, we generated transgenic Arabidopsis lines expressing RWPRK-VP80 using the 4 × NRE-min-GUS line [28] . Differing from the expression of NLP6-VP16, the expression of RWPRK-VP80 led to the constitutive activation of NRE-dependent transcription independently of nitrate treatment ( Fig. 3c ). Thus, the DNA-binding activity of the RWP-RK domain is unrelated to nitrate signalling. 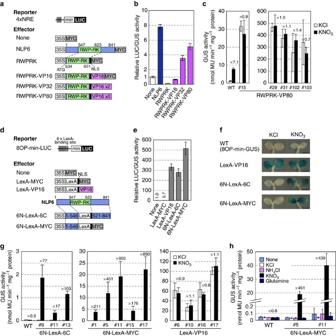Figure 3: The N-terminal region of NLP6 mediates nitrate signalling. (a) A reporter construct and effector constructs used to express the RWP-RK domain of NLP6 fused to multiple copies of the VP16 activation domain. Each construct contained the NOS terminator (not shown). (b) Protoplast transient assays using the reporter and effector constructs shown ina. An internal control plasmid (UBQ10-GUS) was used to normalize the LUC reporter activity levels. (c) GUS activity in the 4 × NRE-min-GUS seedlings (WT) and five independent lines expressing RWPWK-VP80. (d) The reporter construct in which the 8OP promoter was fused to theLUCreporter gene and effector constructs for LexA fusions. (e) Protoplast transient assays with reporter and effector constructs shown ind. Relative LUC activity is shown using GUS activity originating from an internal control plasmid (UBQ10-GUS). (f) GUS staining of KCl-control treated or nitrate-treated seedlings expressing the indicated LexA-fusion proteins. As the background line was 8OP-min-GUS, which harbours theGUSgene under the control of the 8OP promoter, this line is indicated by ’WT‘. Scale bar, 0.5 mm. (g) GUS activity of seedlings expressing LexA fusions. (h) Nitrate-specific induction of GUS activity in seedlings expressing 6N-LexA-MYC. Seedlings of several independent transgenic lines were grown on nitrogen-free medium, treated with 10 mM KCl or KNO3for 4 h and then analysed (c,f,g) or treated with 10 mM KCl, NH4Cl, KNO3or glutamine for 4 h (h). Values are the mean±s.d. (n=3) in (b,c,e,g,h). Induction folds of GUS activity by nitrate treatment are also indicated in (c,g,h). Figure 3: The N-terminal region of NLP6 mediates nitrate signalling. ( a ) A reporter construct and effector constructs used to express the RWP-RK domain of NLP6 fused to multiple copies of the VP16 activation domain. Each construct contained the NOS terminator (not shown). ( b ) Protoplast transient assays using the reporter and effector constructs shown in a . An internal control plasmid (UBQ10-GUS) was used to normalize the LUC reporter activity levels. ( c ) GUS activity in the 4 × NRE-min-GUS seedlings (WT) and five independent lines expressing RWPWK-VP80. ( d ) The reporter construct in which the 8OP promoter was fused to the LUC reporter gene and effector constructs for LexA fusions. ( e ) Protoplast transient assays with reporter and effector constructs shown in d . Relative LUC activity is shown using GUS activity originating from an internal control plasmid (UBQ10-GUS). ( f ) GUS staining of KCl-control treated or nitrate-treated seedlings expressing the indicated LexA-fusion proteins. As the background line was 8OP-min-GUS, which harbours the GUS gene under the control of the 8OP promoter, this line is indicated by ’WT‘. Scale bar, 0.5 mm. ( g ) GUS activity of seedlings expressing LexA fusions. ( h ) Nitrate-specific induction of GUS activity in seedlings expressing 6N-LexA-MYC. Seedlings of several independent transgenic lines were grown on nitrogen-free medium, treated with 10 mM KCl or KNO 3 for 4 h and then analysed ( c , f , g ) or treated with 10 mM KCl, NH 4 Cl, KNO 3 or glutamine for 4 h ( h ). Values are the mean±s.d. ( n =3) in ( b , c , e , g , h ). Induction folds of GUS activity by nitrate treatment are also indicated in ( c , g , h ). Full size image On the other hand, engineered transcription factors in which an Escherichia coli DNA-binding protein LexA [35] was fused to both N- and C-terminal regions of NLP6 (6N-LexA-6C), the N-terminal region alone (6N-LexA-MYC), or the VP16 transcriptional activation domain (LexA-VP16), were found to show comparable activity in protoplasts in terms of the transactivation of the 8OP promoter, which contained eight copies of LexA-binding sites (8OP) upstream of the 35S minimal promoter ( Fig. 3d ). However, these proteins expressed under the control of the 35S promoter differently activated the 8OP promoter in planta . LexA-VP16 elevated GUS expression independently of nitrate treatment, while 6N-LexA-6C or 6N-LexA-MYC strongly induced GUS expression only when the seedlings were treated with nitrate ( Fig. 3f ). Furthermore, unlike nitrate, neither glutamine, a downstream product of nitrate assimilation, nor ammonium activated 6N-LexA-MYC ( Fig. 3h ). These results provide compelling evidence that the N-terminal region flanking the RWP-RK domain is responsible for the activation of NLP6 in response to nitrate signalling. Phenotypic effects of suppression of NLP function The effects of repressing NLP function in planta were investigated through the forced expression of a chimeric repressor, NLP6, fused to the transcriptional repression domain of SUPERMAN [36] (NLP6-SUPRD) ( Fig. 4a ). This construct was chosen because the nine NLPs of Arabidopsis likely have a degree of functional redundancy and NLP6-SUPRD could act as a strong transcriptional repressor of NRE-dependent transcription in protoplasts ( Supplementary Fig. S4 ). Utilization of chimeric repressors is an established and effective approach to investigating the loss of function phenotypes of transcription activators when they have a degree of functional redundancy with other related proteins [37] , [38] , [39] , [40] , [41] . Transgenic Arabidopsis lines expressing NLP6-SUPRD were generated by transformation of the 4 × NRE-min-GUS line [28] (WT in Fig. 4b–e , Supplementary Figs S5,S6 ). The generated lines showed inhibited growth on medium containing nitrate as the sole nitrogen source, as did the NR mutant [42] ( Fig. 4b ). Unlike the NR mutant, however, the NLP6-SUPRD lines showed inhibited growth even on medium containing ammonium. Furthermore, these lines formed smaller rosettes and shorter flowering stems ( Fig. 4d ). These results imply that the expression of NLP6-SUPRD may affect not only the nitrate assimilation process but also other nitrate-responsive processes, reflecting the fact that nitrate signalling is involved in the regulation of various physiological and developmental events [1] , [2] , [9] , [10] . 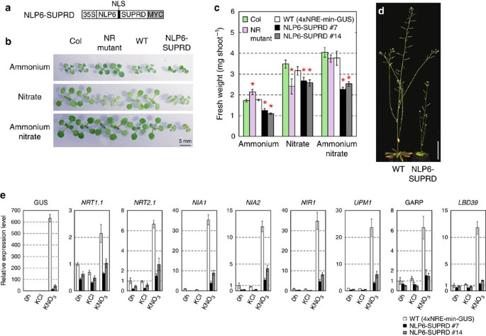Figure 4: Effects of the repression of NLP function. (a) The construct used for the expression of NLP6 fused to a transcriptional repression domain (NLP6-SUPRD). (b,c) Images (b) and fresh weights (c) of wild-type seedlings (Col), the NR mutant, the 4 × NRE-min-GUS line (WT) and the line expressing NLP6-SUPRD, all grown on media containing the indicated nitrogen source for 9 days. Scale bar, 5 mm. Inc, values are the means±s.d. (n=3) and statistical differences from wild-type (two-tailed Student’st-test,P<0.05) are indicated by asterisks. (d) Arabidopsis plant expressing NLP6-SUPRD grown in soil for 45 days. Scale bar, 5 cm. (e) Impaired nitrate-inducible gene expression in the transgenic lines expressing NLP6-SUPRD. The transcript levels of GUS, as well as typical nitrate-inducible genes were analysed using seedlings of the 4 × NRE-min-GUS line (WT) and two independent NLP6-SUPRD lines. Seedlings grown in medium containing ammonium as the sole nitrogen source were treated with 10 mM KCl or KNO3for 1 h.NRT1;1, a dual-affinity nitrate transporter gene;NRT2;1, a high-affinity nitrate transporter gene;NIA1andNIA2, nitrate reductase genes;NIR1, nitrite reductase gene;UPM1, uroporphyrin-III C-methyltransferase gene; GARP, a GARP-type transcription factor gene (At1g25550);LBD39, a LBD domain-containing protein gene. Values are the means±s.d. (n=3). Figure 4: Effects of the repression of NLP function. ( a ) The construct used for the expression of NLP6 fused to a transcriptional repression domain (NLP6-SUPRD). ( b , c ) Images ( b ) and fresh weights ( c ) of wild-type seedlings (Col), the NR mutant, the 4 × NRE-min-GUS line (WT) and the line expressing NLP6-SUPRD, all grown on media containing the indicated nitrogen source for 9 days. Scale bar, 5 mm. In c , values are the means±s.d. ( n =3) and statistical differences from wild-type (two-tailed Student’s t -test, P <0.05) are indicated by asterisks. ( d ) Arabidopsis plant expressing NLP6-SUPRD grown in soil for 45 days. Scale bar, 5 cm. ( e ) Impaired nitrate-inducible gene expression in the transgenic lines expressing NLP6-SUPRD. The transcript levels of GUS, as well as typical nitrate-inducible genes were analysed using seedlings of the 4 × NRE-min-GUS line (WT) and two independent NLP6-SUPRD lines. Seedlings grown in medium containing ammonium as the sole nitrogen source were treated with 10 mM KCl or KNO 3 for 1 h. NRT1;1 , a dual-affinity nitrate transporter gene; NRT2;1 , a high-affinity nitrate transporter gene; NIA1 and NIA2 , nitrate reductase genes; NIR1 , nitrite reductase gene; UPM1 , uroporphyrin-III C-methyltransferase gene; GARP, a GARP-type transcription factor gene (At1g25550); LBD39 , a LBD domain-containing protein gene. Values are the means±s.d. ( n =3). Full size image Suppression of NLP downregulates nitrate-inducible genes We also investigated the effects of expressing NLP6-SUPRD on nitrate-inducible gene expression using two independent NLP6-SUPRD lines ( Fig. 4e ). The expression of typical nitrate-inducible genes, including two major nitrate transporter genes ( NRT1;1 and NRT2;1 ), nitrate assimilation-related enzyme genes ( NIA1 , NIA2 , NIR1 and UPM1 ) and transcription factor genes (a GARP-type transcription factor gene and LBD39 ), was analysed. In the NLP6-SUPRD lines, the nitrate-inducible expression of all analysed genes, as well as NRE-dependent GUS expression was severely diminished, suggesting that NLP activity is responsible for the expression of most nitrate-inducible genes. Importantly, severe reductions in the expression of transcription factor genes suggest that NLP can induce a broad outcome through transcriptional cascades. Unexpectedly, the growth of the NLP6-SUPRD lines showed a slight but statistically significant decrease in growth even on medium containing ammonium as the sole nitrogen source ( Fig. 4b ). A possible explanation of this phenomenon is that because the DNA-binding activity of NLPs is independent of nitrate signalling, NLP6-SUPRD binds to its target sites and reduces the basal expression levels of the NLP target genes even in the absence of nitrate. Indeed, in agreement with this hypothesis, reductions in the basal expression levels of the genes involved in nitrate uptake or reduction were found in the NLP6-SUPRD lines ( Fig. 4e ). We, therefore, speculated that such reductions in the expression of genes that are not involved in nitrate utilization but other growth-related processes might lead to a decrease in the growth of the NLP6-SUPRD lines even on ammonium medium. By investigation of the expression levels of ammonium assimilation-related enzyme genes in the NLP6-SUPRD lines, both the basal and nitrate-induced expression levels of the chloroplastic glutamine synthetase gene ( GLN2 ) [9] , [43] were found to be reduced in the NLP6-SUPRD lines ( Supplementary Fig. S6 ). Thus, the NLP function is likely involved in regulating the expression of not only genes for nitrate uptake or reduction but also genes that function in other metabolic processes. Here we report that NLP6 and probably other NLPs are nitrate-responsive transcription factors which primarily respond to nitrate signals and convert them to transcriptional control events in Arabidopsis ( Fig. 5 ). This finding is the key to the understanding of the molecular basis of nitrate-regulated gene expression in higher plants. Despite the nomenclature of NLPs, which was assigned on the basis of their similarity to NIN protein, it should be noted that the NLP family of proteins was originally associated with nitrate-regulated gene expression, because such gene expression occurs throughout the plant kingdom, whereas symbiotic nitrogen fixation is unique to leguminous plants. NIN is likely a variant of NLP, which evolved specifically for symbiotic nitrogen fixation in legumes. 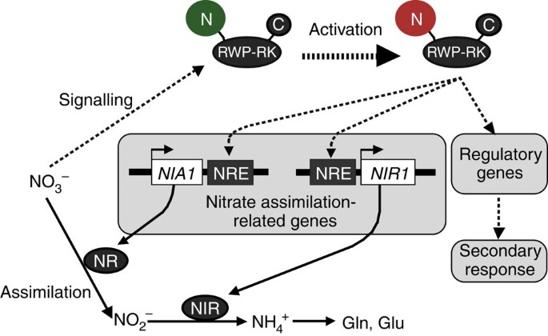Figure 5: A model for NLP function in the nitrate response pathway. The nitrate signal transmitted through its signalling pathway converts the inactive form of the N-terminal regions of NLPs into active forms, which are indicated in green and red, respectively. Post-translationally activated NLPs promote the expression of nitrate-inducible genes through interaction with NREs. As NLPs activate both the genes involved in nitrate assimilation and regulatory genes including transcription factor genes, the nitrate-induced activation of NLPs can produce a broad range of regulatory outcomes. Figure 5: A model for NLP function in the nitrate response pathway. The nitrate signal transmitted through its signalling pathway converts the inactive form of the N-terminal regions of NLPs into active forms, which are indicated in green and red, respectively. Post-translationally activated NLPs promote the expression of nitrate-inducible genes through interaction with NREs. As NLPs activate both the genes involved in nitrate assimilation and regulatory genes including transcription factor genes, the nitrate-induced activation of NLPs can produce a broad range of regulatory outcomes. Full size image Our results suggest that nitrate signal converts an inactive form of NLPs into an active form ( Fig. 3 ) that can bind to NREs within the NIR1 and NIA1 loci ( Fig.1 and Supplementary Fig. S1a,b ) and promote the expression of these genes. This further suggests that the post-translational activation of NLPs may be a key step in the transmission of signals from the nitrate signalling pathway to transcriptional control mechanisms ( Fig. 5 ). NLPs were also found to modulate the expression of other major genes associated with nitrate transport or nitrogen assimilation processes ( Fig. 4d , Supplementary Fig. S6 ). Furthermore, our findings that the expression of LBD39 (ref. 21 ) and a GARP-type transcription factor gene [10] are also under the control of NLPs ( Fig. 4d ) indicate that NLP functions include the regulation of nitrate-inducible regulatory factor genes, which would produce a broad range of regulatory outcomes. We have not yet identified NLP-binding sites other than those at NIR1 and NIA1 loci. However, these genes, which were found to be downregulated in the NLP6-SUPRD lines, are probably direct target genes of NLPs because they are all nitrate-inducible in a sensitive and prompt manner. These findings strongly suggest that NLPs have a central role in the nitrate response via the regulation of the nitrate-inducible expression of many genes, including metabolic enzyme genes and regulatory factor genes. Based on the findings, we propose a model for the NLP-mediated regulation of the nitrate response ( Fig. 5 ). Although it is still arguable that all Arabidopsis NLPs mediate nitrate signals and have any role in the nitrate response pathways, we postulate that most NLPs may be involved in nitrate-induced gene expression. In the case of some transcription factor families, such as the auxin response factor and response regulator type B families that are involved in auxin and cytokinin signalling pathways, respectively [44] , [45] , each family member has overlapping and/or unique roles to respond to the particular stimulus. Similarly, individual NLPs may have overlapping and/or unique roles in the nitrate response. This hypothesis is supported by our evidence that the RWP-RK domains of all of the NLPs we tested bind to the NRE in vitro ( Fig. 1b ) and that the NRE-containing promoter is transactivated by each of the NLPs tested in vivo ( Fig. 2a ). This hypothesis is also in agreement with the reported reductions in the nitrate-inducible expression of NR and nitrate transporter genes in nlp7 mutants [19] . Furthermore, we have shown that the N-terminal region of NLP6, which had high homology to that of other Arabidopsis NLPs [31] , functions as a nitrate-responsive domain ( Fig. 3 ), implying that all Arabidopsis NLPs may be activated by nitrate through their conserved amino-acid sequences. However, because we also found similar but not identical binding specificity of the RWP-RK domains of Arabidopsis NLPs ( Fig. 1d ), further analysis of interactions between each NLP with NREs of various nitrate-induced genes, as well as analysis of temporal and spatial expression patterns of each NLP gene will be necessary in the future to clarify the physiological relevance of each NLP to the nitrate response network. From the results in our current study, new and important questions regarding the mechanisms for the nitrate response have emerged. The first of these is how nitrate signalling converts an inactive form of NLP into its active counterpart post-translationally. The second is how plant cells sense nitrate signals and transmit then to the regulatory mechanisms for NLP activity. As the 6N-LexA-6C and 6N-LexA-MYC constructs did not transactivate the 8OP promoter at all without nitrate treatment in the transgenic seedlings ( Fig. 3f–h ), whereas they could do so in protoplasts prepared from mature leaves ( Fig. 3e ), the post-translational activation of NLPs appears to occur in response to endogenous nitrate in protoplasts. This possibility needs to be carefully examined in future studies. A third major mechanistic question is how many and what kinds of genes are under the direct or indirect control of NLPs. Although our present results have already suggested that the nitrate-inducible expression of a series of genes for nitrate transport and assimilation, as well as transcription factor genes, is regulated by NLPs, a larger number of genes are likely to be controlled by NLP activity. Comprehensive analysis of NLP target genes and NLP-binding sites on the genome would likely clarify the central role of NLPs in the nitrate response system in higher plants. Y1H screening Reporter plasmids, p4 × NRE-HIS and p4 × NRE(M2)-HIS, were constructed by inserting four copies of the wild-type or mutated NRE between the Eco RI and Xba I sites of pHISi-1 and then used to transform the yeast strain YM4271 (Matchmaker One-Hybrid System; Clontech Laboratories, Inc). Arabidopsis cDNA were generated using RNA from 3-week-old leaves of wild-type Arabidopsis (ecotype Columbia) and random or oligo-dT primers. The cDNA, together with linearized pGAD-T7-Rec vector (Matchmaker Gold Yeast One-Hybrid Library Screening System), were used to transform yeast harbouring the 4 × NRE-HIS reporter gene. Transformants were grown on SD-Leu-His plates containing 15 mM 3-aminotriazole for 7 or 8 days at 26 °C for selection. For confirmation of the results, cDNAs encoding the RWP-RK domain of Arabidopsis NLPs were newly amplified by PCRs with cDNA libraries and then cloned into the pGAD-T7 vector (Clontech Laboratories, Inc). Yeast harbouring 4 × NRE-HIS or 4 × NRE(M2)-HIS reporter genes were transformed using the resultant plasmids. The primers used for cDNA cloning are listed in Supplementary Table S2 . Electrophoretic mobility shift assay DNA fragments encoding the RWP-RK domain were subcloned into pET32 (Merck Biosciences). His-tagged recombinant proteins were expressed in E. coli using resultant vectors and purified using Ni-NTA resin (His·Bind resin, Novagen) according to the manufacturer’s protocol. EMSA were performed as described previously [46] . Briefly, a 5′-biotinylated probe was generated by PCR with 5′-end biotinylated primers. Recombinant proteins (75 ng) were mixed with the 2.5 ng of biotin-labelled DNA probe in a buffer containing 0.5 μg poly [d(I-C)], 20 mM HEPES-KOH (pH 7.6), 3 mM MgCl 2 , 2 mM dithiothreitol, 0.5 mM EDTA, 30 mM KCl, 30 mM NaCl and 10% glycerol, and then incubated at room temperature for 30 min. The reaction mixtures were subjected to electrophoresis in native 5% polyacrylamide gels in 0.5 × TBE. The DNA in the gel was then transferred onto positively charged nylon membranes (Biodyne B, PALL). The DNA on the membranes was detected using streptavidin-conjugated horseradish peroxidase (Pierce). Plant growth conditions For quantitative reverse transcription PCR (RT–PCR) analysis of nitrate-inducible expression, seeds were stratified in nitrogen-free 1/2MS medium (half-strength MS salts from which ammonium nitrate and potassium nitrate were eliminated, Gamborg’s B5 vitamin mixture, and 0.5 g l −1 MES (pH 5.7)) for 3 days and then incubated under continuous light at 23 °C for germination and seedling growth. After 3.5 days, the medium was changed to fresh nitrogen-free 1/2MS liquid medium supplemented with various concentrations of KNO 3 . To analyse the induction of GUS activity by nitrate, seeds were sown on agar plates containing nitrogen-free 1/2MS medium supplemented with 0.5% sucrose. After stratification, the plates were placed vertically at 23 °C under continuous light for 3.5 days and 1 ml of 10 mM KCl or KNO 3 solution was then applied. The plates were placed horizontally and incubated for 4 h before collecting shoots for the GUS assay. For phenotypic analysis, the transgenic lines expressing NLP6-SUPRD were grown together with wild-type Arabidopsis (Columbia), an NR mutant (G′4-3) [42] and the 4 × NRE-min-GUS line (line #1) [28] on nitrogen-free 1/2MS agar plates supplemented with 1% sucrose and either 5 mM KNO 3 , 5 mM NH 4 NO 3 or 2.5 mM ammonium succinate. When ammonium succinate was supplied as the nitrogen source, the pH of the medium was adjusted to 6.5. For the preparation of mesophyll protoplasts, Arabidopsis (Columbia) were grown on peat containing nutrients (Sakatanotane Co., Yokohama, Japan) at 23 °C for 3 weeks under continuous light. Protoplast transient assay For the construction of effector plasmids to express NLPs, EIN3 cDNA in the 35SC4PPDK-EIN3-MYC construct [34] was replaced with NLP cDNAs. To construct effector plasmids to express NLP6-VP16 and RWPRK-VP16 proteins, the sequences for LexA and GR in the 35SC4PPDK-LexA-NLS-VP16-GR construct [34] were replaced with NLP6 cDNA or the sequence encoding the RWP-RK domain of NLP6 and the sequence for a MYC-tag, respectively. The MYC-tag sequence of a resultant construct, 35SC4PPDK- RWPRK, was replaced with the sequence encoding one or four copies of the VP16 transcriptional activation domain to generate effector plasmids to express RWPRK-VP32 and -VP80. On the other hand, the sequence for the VP16 transcriptional activation domain in another resultant construct, 35SC4PPDK-NLP6-VP16, was replaced with the sequence for a repressor domain of SUPERMAN (175–204 amino acids) to generate an effector plasmid for the expression of NLP6-SUPRD. Similarly, effector plasmids that express LexA fusions were generated. The effector plasmid for the expression of LexA alone was initially constructed by the replacement of EIN3 cDNA in the 35SC4PPDK-EIN3-MYC construct with the sequence encoding LexA and a nuclear localization signal. Using the obtained plasmid, expression vectors for 6N-LexA-MYC and 6N-LexA-6C proteins were generated. The sequence for the N-terminal region (1–546 amino acids) of NLP6 was inserted between the 35SC4PPDK promoter and the LexA coding region to produce the expression vector for the 6N-LexA-MYC protein. Subsequently, the plasmid used to express the 6N-LexA-6C protein was produced by replacement of the MYC-tag sequence with the sequence encoding the C-terminal region of NLP6 (621–841 amino acids). Reporter plasmids that contained the LUC reporter gene downstream of the wild-type or mutated NIR1 promoter were constructed using the 1.27 kb DNA fragment for the wild-type and mutated NIR1 promoters [28] . The promoters were substituted for the 35S promoter in pJD301 (ref. 47 ). As our plasmid construction was performed using DNA fragments, which were obtained by PCR amplification using the primers listed in Supplementary Table S2 , all constructs were verified by DNA sequencing. Mesophyll protoplasts were isolated from rosette leaves. A reporter (6 μg) and an effector plasmid (12 μg) were co-transfected together with an internal control plasmid (UBQ10-GUS; 2 μg) into 2 × 10 4 protoplasts by a polyethylene glycol-mediated transfection method [33] . Transfected protoplasts were incubated overnight at 23 °C in the dark in the absence of exogenous nitrate and then lysed with Cell Culture Lysis Solution (Promega). Measurements of LUC and GUS activity with cell lysate were performed with a Luciferase Assay System kit (Promega) and a fluorescent substrate, 4-methylumbelliferyl-β-D-glucuronide, respectively [34] . Relative LUC activity was calculated performed with obtained values [34] . Generation of transgenic lines For the construction of binary vectors to generate transgenic Arabidopsis expressing NLP6-VP16, RWPRK-VP80 or NLP6-SUPRD under the control of the 35S promoter, we initially generated a binary vector pCB302-HYG-35S-GUS, which was generated by replacing the bar gene in pCB302-35S-GUS [48] with a hygromycin resistance gene. The GUS gene was then replaced with DNA fragments encoding either NLP6-VP16, RWPRK-VP80 or NLP6-SUPRD. Using these constructed binary vectors, the 4 × NRE-min-GUS line (line #1) [28] was transformed with the floral dip method. Transgenic Arabidopsis harbouring the GUS reporter gene under the control of the 8OP promoter was generated by transformation of wild-type Arabidopsis (Columbia) using a binary vector where the 35S promoter in pCB302-HYG-35S-GUS was replaced with the 8OP promoter. Transgenic Arabidopsis lines expressing LexA fusions were produced by retransformation of the transgenic Arabidopsis plants with binary vectors for the expression of LexA-MYC, LexA-VP16, 6N-LexA-MYC or 6N-LexA-6C under the control of the 35S promoter, which were constructed by replacement of the GUS gene in pCB302-35S-GUS [48] with DNA fragments encoding either LexA-MYC, LexA-VP16, 6N-LexA-MYC or 6N-LexA-6C. Quantitative reverse transcription PCR RNA preparation and qRT-PCR were performed as described previously [28] . Briefly, reverse transcription were performed with SuperScript II reverse transcriptase (Invitrogen) and the oligo-dT primer, and PCR reactions were performed with a StepOne Plus Real Time PCR System (Applied Biosystems) using the KAPA SYBR Fast quantitative PCR Kit (KAPA Biosystems). The primers used are listed in Supplementary Table S2 . GUS staining and measurements of transgenic plants For histochemical GUS staining, seedlings were fixed in ice-cold 90% acetone, rinsed in 0.1 M NaPO 4 buffer (pH7.4) and incubated in X-Gluc buffer (0.1 M NaPO 4 (pH7.4), 0.5 mM potassium ferricyanide, 0.5 mM potassium ferrocyanide, 0.5 mg ml −1 5-bromo-4-chloro-3-indolyl-β- D -glucuronide cyclohexylammonium salt) at 37 °C [28] , [48] . Stained samples were observed under a stereomicroscope (MZ16F, Leica Microsystems, Germany) and photographed with a DXM1200C digital camera (Nikon, Japan). Measurements of GUS activity were performed as described previously [28] . The shoots were homogenized in extraction buffer (50 mM NaPO 4 (pH 7.4), 10 mM EDTA, 0.1% Triton X-100, 0.1% sodium lauryl sarcosine, 10 mM β-mercaptoethanol), and enzyme reactions were carried out with the extract in the extraction buffer containing 1 mM 4-methylumbelliferyl-β- D -glucuronide. Fluorescence of released 4-methylumbelliferone was measured using the Infinite M1000 microplate reader (TECAN Group Ltd). How to cite this article: Konishi, M. et al . Arabidopsis NIN-like transcription factors have a central role in nitrate signalling. Nat. Commun. 4:1617 doi: 10.1038/ncomms2621 (2013).